Rechargeable aqueous zinc-manganese dioxide batteries with high energy and power densities Although alkaline zinc-manganese dioxide batteries have dominated the primary battery applications, it is challenging to make them rechargeable. Here we report a high-performance rechargeable zinc-manganese dioxide system with an aqueous mild-acidic zinc triflate electrolyte. We demonstrate that the tunnel structured manganese dioxide polymorphs undergo a phase transition to layered zinc-buserite on first discharging, thus allowing subsequent intercalation of zinc cations in the latter structure. Based on this electrode mechanism, we formulate an aqueous zinc/manganese triflate electrolyte that enables the formation of a protective porous manganese oxide layer. The cathode exhibits a high reversible capacity of 225 mAh g −1 and long-term cyclability with 94% capacity retention over 2000 cycles. Remarkably, the pouch zinc-manganese dioxide battery delivers a total energy density of 75.2 Wh kg −1 . As a result of the superior battery performance, the high safety of aqueous electrolyte, the facile cell assembly and the cost benefit of the source materials, this zinc-manganese dioxide system is believed to be promising for large-scale energy storage applications. There is ever increasing demand of advanced battery technologies with high safety and low cost for applications in portable electronics, electrified vehicles, and renewable energy storage [1] , [2] , [3] , [4] , [5] , [6] , [7] . Although lithium-ion batteries have gained great improvement in energy/power density and life span, the safety issues associated with flammable organic electrolytes and the growing concerns of the price and availability of Li resources impede their large-scale deployment. Battery chemistries based on electrochemical intercalation/storage of Na + , K + , Mg 2+ , and Zn 2+ in aqueous electrolytes have been considered as promising alternatives, because of high safety, materials abundance, and environmental friendliness [8] , [9] , [10] , [11] , [12] , [13] , [14] , [15] , [16] , [17] , [18] , [19] . Rechargeable Zn-ion batteries (ZIBs) are particularly attractive as zinc features higher water compatibility and stability than alkaline metals, allows multivalent charge transport carriers, and can be produced and recycled with mature industrial process [20] , [21] , [22] , [23] , [24] , [25] . Zinc-manganese dioxide (Zn-MnO 2 ) batteries have dominated the primary battery market because of low cost, high safety, and easy manufacturing [26] , [27] , [28] . It is highly intriguing to develop rechargeable Zn-MnO 2 batteries. Nevertheless, previous attempts are plagued by poor cycling performance due to the formation of irreversible discharged species (e.g., Mn(OH) 2 and ZnO at cathode and anode, respectively) in alkaline electrolytes [29] , [30] , [31] . Although alkaline Zn-MnO 2 batteries (Fig. 1a ) were shown rechargeable for extended cycles, the delivered capacity is limited at shallow depth of discharge (~ 10%) [32] . Recently, the rechargeability of aqueous Zn-MnO 2 batteries has been improved by using mild acidic electrolyte (e.g., aqueous ZnSO 4 solution) [33] − [37] . However, the reaction mechanism of MnO 2 polymorphs remains elusive and controversial. For example, electrochemical Zn-insertion in α-MnO 2 is shown to undergo phase transition from tunneled structure to spinel ZnMn 2 O 4 [33] , layered Zn-buserite [36] , or birnessite [38] , most of which collapse upon cycling. A different mechanism was referred to the conversion reaction between α-MnO 2 and MnOOH [35] . For γ-MnO 2 , complex mutiple-phase transformation was proposed on discharge, involving spinel-type ZnMn 2 O 4 , tunnel-type γ-Zn x MnO 2 , and layered-type L-Zn x MnO 2 [34] . Additionally, the Zn-insertion properties in aqueous ZnSO 4 electrolyte are found to vary among polymorphs: α-MnO 2 featuring (2 × 2) + (1 × 1) tunnel structure [39] and γ-MnO 2 with (1 × 2) + (1 × 1) tunnels exhibit high capacity (150‒300 mAh g −1 ) [34] , [36] , whereas the most stable (1 × 1) tunneled β-MnO 2 phase [40] , [41] hardly incorporates Zn 2+ ions [33] due to narrow tunnels [42] . Furthermore, in the widely investigated ZnSO 4 electrolyte, MnO 2 generally suffers from capacity loss due to the dissolution of Mn 2+ from Mn 3+ disproportionation [34] , [35] . Pre-addition of Mn 2+ salt is proposed to improve capacity retention [35] but the underneath mechanism remains unclear. Our previous study indicates that the use of zinc salt with bulky anion (e.g., CF 3 SO 3 − ) benefits reactivity and stability of Zn anode and spinel ZnMn 2 O 4 cathode [24] . Therefore, elucidating the electrode reactions of MnO 2 and exploiting compatible electrolyte are desirable in developing rechargeable aqueous Zn-MnO 2 batteries. Fig. 1 Zn-MnO 2 battery chemistry. Schematic illustration of a the primary alkaline Zn-MnO 2 battery using KOH electrolyte and b the rechargeable Zn-MnO 2 cell using CF 3 SO 3 − -based electrolyte. c Comparison of the cycling performance of Zn-MnO 2 cells with electrolytes of 45wt.% KOH (at 0.32 C), 3 M ZnSO 4 , 3 M Zn(CF 3 SO 3 ) 2 , and 3 M Zn(CF 3 SO 3 ) 2 with 0.1 M Mn(CF 3 SO 3 ) 2 additive at 0.65 C. n C equals the rate to charge/discharge the thereotical capacity (308 mAh g −1 ) of MnO 2 in 1/ n hours Full size image Herein, we report high-performance rechargeable aqueous Zn-MnO 2 cells based on MnO 2 cathode, Zn anode, and Zn(CF 3 SO 3 ) 2 electrolyte with Mn(CF 3 SO 3 ) 2 additive. For the widely investigated α-, β-, and γ-MnO 2 polymorphs, we elucidate a common electrode reaction mechanism, by combining electrochemical measurements, X-ray diffraction analysis (XRD), elemental analysis, transmission electron microscopy (TEM), and synchrotron X-ray absorption spectroscopy (XAS). Interestingly, in the exemplified β-MnO 2 that has been previously demonstrated unfavorable for Zn intercalation, a layer-type phase (i.e., Zn-buserite B-Zn x MnO 2 · n H 2 O) is generated during the initial discharge, followed by reversible insertion/extraction of Zn 2+ ions in the layered structure (Fig. 1b ). Up to ~ 0.5 Zn per molecular MnO 2 is accommodated on discharging, along with disproportionated Mn dissolution and capacity fade. We significantly improve the cycling stability of Zn-MnO 2 cell by employing concentrated Zn(CF 3 SO 3 ) 2 electrolyte and Mn(CF 3 SO 3 ) 2 additive (Fig. 1c ). The pre-added Mn(CF 3 SO 3 ) 2 is found to suppress Mn 2+ dissolution and result in the formation of a uniform porous MnO x nanosheet layer on the cathode surface, which helps to maintain the electrode integrity. Remarkably, β-MnO 2 exhibits high reversible capacity, high rate capability, and stable cyclability. We further demonstate a soft-packed Zn-MnO 2 full cell that delivers a reversible capacity of 1550 mAh with a total energy density of 75.2 Wh kg −1 after 50 cycles. Materials synthesis and characterization We selected pyrolusite β-MnO 2 as a model polymorph, which has been previously demonstrated to exhibit extremely poor electrochemical activity [33] and was prepared by a simple hydrothermal route in this study (detailedly described in experimental section). X-ray diffraction patterns (XRD, Supplementary Fig. 1a ) reveals high purity of the formed tetragonal phase (JCPDS no. 24-735) with P42/mnm space group. Scanning electron microscope (SEM, Supplementary Fig. 1b ) of the sample displays nanorod morphology with average length of 2 μm and width of 100–200 nm. Polymorphs of α-MnO 2 and γ-MnO 2 nanorods were also synthesized via hydrothermal technique (Supplementary Fig. 2 ; Supplementary Methods ). Commerical β-MnO 2 powders with large particle size of ~ 2 μm (Supplementary Fig. 3 ) were employed for comparison. Electrode reaction mechanism Figure 2a shows the cyclic voltammograms (CVs) of β-MnO 2 in aqueous 3 M Zn(CF 3 SO 3 ) 2 electrolyte. 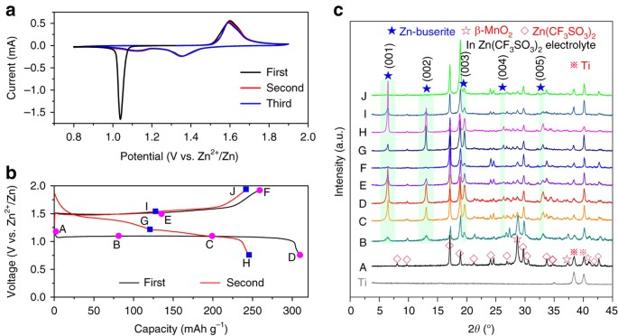Fig. 2 Electrochemical and structural evolution of β-MnO2in Zn-MnO2cell.aCyclic voltammograms of β-MnO2electrode at a scan rate of 0.1 mV s−1from 0.8 to 1.9 V.bTypical charge/discharge curves for the initial two cycles at 0.32 C in 3 M Zn(CF3SO3)2aqueous electrolyte. The points A–J marked the states where data were collected for XRD analysis.cXRD patterns of β-MnO2electrode at selected states during the first and second cycles A sharp peak at around 1.06 V is observed during the first cathodic sweeping. In the following cycles, the CV curves are well repeated with two cathodic peaks located at 1.35 and 1.17 V and an overlapped anodic peak at 1.6/1.65 V. The significant difference in CV profiles between the initial and subsequent cycles suggests phase transition. Figure 2b shows the typical galvanostatic profiles of β-MnO 2 at 0.32 C. The first discharge curve displays a flat plateau at around 1.08 V while the second cycle presents two slopping discharge plateaus, in line with the CV results. Notably, the initial discharge capacity reaches 307 mAh g −1 , which approaches the theoretical capacity of 308 mAh g −1 (based on MnO 2 ) and corresponds to 0.5 Zn 2+ per MnO 2 . The evolution of CV profiles and discharge plateaus indicates different mechanism of Zn 2+ intercalation in MnO 2 electrode [36] , [43] , as discussed below. Fig. 2 Electrochemical and structural evolution of β-MnO 2 in Zn-MnO 2 cell. a Cyclic voltammograms of β-MnO 2 electrode at a scan rate of 0.1 mV s −1 from 0.8 to 1.9 V. b Typical charge/discharge curves for the initial two cycles at 0.32 C in 3 M Zn(CF 3 SO 3 ) 2 aqueous electrolyte. The points A–J marked the states where data were collected for XRD analysis. c XRD patterns of β-MnO 2 electrode at selected states during the first and second cycles Full size image To probe the structural evolution of β-MnO 2 in the discharge/charge process, ex-situ XRD patterns (Fig. 2c ) were recorded at the selected states (marked points in Fig. 2b ). On first discharging (A → D), the characteristic peaks of β-MnO 2 are gradually weakened and new phase arises. Besides the peaks designated to the Zn(CF 3 SO 3 ) 2 salt, new peaks emerge at 6.47, 13.00, 19.58, 26.28, and 32.93°, which could be assigned to reflections from the (001)–(005) crystallographic planes of a layered Zn-buserite phase, respectively. The electrolyte salt is precipitated on the surface of both MnO 2 cathode and Zn anode but can be easily removed by immersing and rinsing with water (Supplementary Fig. 4a–c ). Notably, the XRD pattern of the rinsed cathode differs from that of previously reported species (e.g., MnOOH [35] , spinel ZnMn 2 O 4 [33] , birnessite [38] , tunneled γ-ZnMnO 2 [34] , and layered L-Zn x MnO 2 [34] ) in discharged MnO 2 electrodes (Supplementary Fig. 4d ). Rietveld refinement of the XRD data of the discharged electrode suggests the formation of Zn-buserite phase (Supplementary Fig. 4e ). The exact structural motif of Zn-buserite is not determined yet, but will be further investigated in the future. The Zn-buserite phase, commonly found in layered Mn oxide mineral [44] , [45] , [46] , contains H 2 O layers in the channels between two MnO 6 octohedron slabs (Fig. 1b ), featuring a similar structure with Ca-buserite [44] (JCPDS No.50-0015). Zn 2+ cations reside above and below the Mn vacant sites and are coordinated with three O atoms adjacent to the vacancies and three O atoms from interlayer H 2 O [36] , [44] , [45] , [46] . The presence of H 2 O in the discharged species was validated using thermal gravimetric analysis (TGA), indicating a composition of ~ 2.28 molecular H 2 O per formula of Zn-buserite (Supplementary Fig. 5 ). In the followed charging process (D→F), the intensity of characteristic peaks for the layered phase was gradually weakened upon extraction of Zn ions. This peak attenuation could be explained by the decrease of scattering atom concentration in unit cell and the weakening of Zn–O interaction due to Zn egress. Similar intensity variation of (00 l ) reflection has been observed on layered intercalation electrodes such as vanadium oxides [9] , [47] . In the second cycle, the signals of layered compound were reversibly strengthened/weakened upon Zn 2+ insertion/extraction. The presence of β-MnO 2 can be observed in the initial several cycles but is not discernable after 10 cycles (Supplementary Fig. 6 ). We investigated the structural evolution of α-MnO 2 and γ-MnO 2 cathodes as well. Interestingly, these two polymorphs undergo phase transformation to layered Zn-buserite upon first discharging and reversible Zn intercalation in the layered structure on subsequent cycling (Supplementary Figs. 7 and 8 ), resembling the case of β-MnO 2 . The results suggest common electrode reaction mechanism in tunneled polymorphs of MnO 2 , which to the best of our knowlege, is first elucidated in mild acidic electrolytes. The structural evolution of β-MnO 2 electrode was further investigated by ex-situ TEM analysis. Figure 3a, b displays the TEM and high-resolution TEM (HRTEM) images at the initial state, where the lattice fringes can be indexed to the (110) plane of β-MnO 2 . 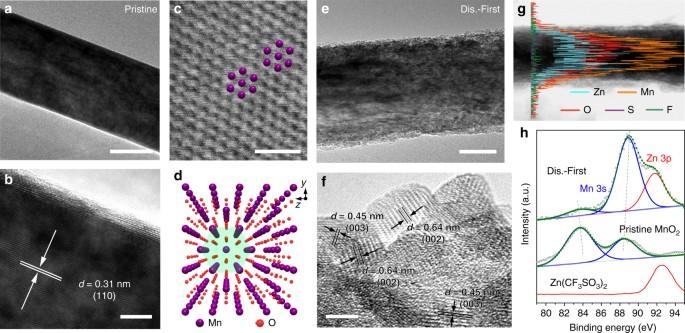Fig. 3 Microstructural and compositional analysis of MnO2.aTEM image,bHRTEM image,cABF-STEM image, anddschematic atomic model (viewed from the [100] zone axis) at the initial state.eTEM image,fHRTEM image,gEDS line scanning profiles in TEM, andhXPS spectra of the first fully discharged electrode.Scale bars, 50 nma,e; 5 nmb,f; and 1 nmc, respectively The annular bright field-scanning TEM (ABF-STEM) image (Fig. 3c ) clearly shows the atomic arrangement within the tunnel-like framework, as schematically viewed along the [100] direction of the lattice (Fig. 3d ). After fully discharging, the one-dimensional nanorod shape is maintained, while the surface of electrode becomes rough with the formation of aggregated nanoparticles (Fig. 3e ), which is ascribed to the structural distortion in the phase-conversion process. The observed lattice fringes with interplanar distances of 0.45, 0.64, and 1.29 nm correspond to the (003), (002), and (001) planes of Zn-buserite (Fig. 3f and Supplementary Fig. 9a ), respectively, consistent with the XRD analysis. Fig. 3 Microstructural and compositional analysis of MnO 2 . a TEM image, b HRTEM image, c ABF-STEM image, and d schematic atomic model (viewed from the [100] zone axis) at the initial state. e TEM image, f HRTEM image, g EDS line scanning profiles in TEM, and h XPS spectra of the first fully discharged electrode. Scale bars , 50 nm a , e ; 5 nm b , f ; and 1 nm c , respectively Full size image To eliminate the impact of precipitated electrolyte salt, the discharged electrode was rinsed with water for elemental dispersive spectroscopy (EDS) and X-ray photoelectron spectroscopy (XPS) analysis. The line scanning profile in TEM (Fig. 3g ) and elemental mapping (Supplementary Fig. 9b ) in STEM of the discharged electrode reveal the uniform distribution of Zn, Mn and O, whereas S and F from electrolyte are not detectable (Fig. 3g ). In XPS spectra, the energy splitting (Δ E ) of Mn 3 s doublet peaks is 4.7 and 5.0 eV for pristine and discharged electrodes, respectively, indicating reduced Mn valence after Zn insertion (Fig. 3h ). At discharged state, a new Zn 3p peak appears at 92.0 eV, which is lower than that of Zn(CF 3 SO 3 ) 2 (92.7 eV) and could be assigned to the intercalated Zn. These results confirm the presence of Zn 2+ ions into the layered manganese oxide host and rule out the possibility of electrode reactions associated with CF 3 SO 3 − anions. Furthermore, the TEM images of β-MnO 2 electrode after different cycles (Supplementary Fig. 10 ) indicate expansion and exfoliation of nanorods, which is attributed to the phase transition, Mn dissolution and repeated Zn 2+ intercalation, and would incur capacity loss during cycling. To gain insight into the variation of Mn oxidation state and electronic structure during the (de)intercalation process, we performed the synchrotron XAS characterization, which has been demonstrated useful to analyze manganese oxides [48] , [49] , [50] , [51] , [52] . Figure 4a shows the normalized Mn K-edge XANES (X-ray near edge absorption structure) profiles of β-MnO 2 electrode at selected states in the initial two cycles. 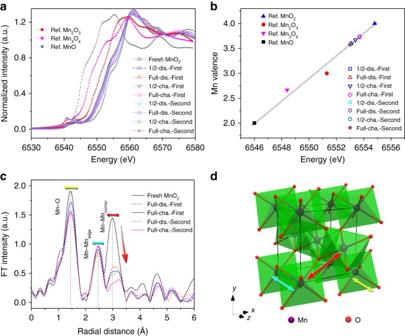Fig. 4 XAS characterization of β-MnO2electrode.aMn-K edge XANES curves at selected discharge/charge states, with reference to standard MnO, Mn2O3,and Mn3O4.bFitted linear relationship between the photon energy and oxidation state of Mn element.cThe EXAFS spectra.dSchematic depiction of the unit cell of β-MnO2 The nominal Mn valence was plotted vs. excitation energy of reference manganese oxides to establish fitted linear correlation (Fig. 4b ). On discharging, the entire edge shifts toward lower energy, indicating a decrease of the average Mn oxidation state. The mean Mn valence at fully discharged state is estimated to be 3.6. During first charging, the edge position slightly shifts back to higher energy, while it remains almost unchanged in the second cycle. The interesting point is that the Mn valence should increase/decrease with Zn 2+ intercalation/deintercalation and would approach 3 for the fully discharged electrode, as anticipated from the discharged capacity (Fig. 2b ). We postulate that such unexpected observation could be ascribed to the disproportional dissolution of trivalent Mn species (Mn 3+ s → Mn 4+ s + Mn 2+ aq ) [38] , [53] . Analysis of Mn by inductively coupled plasma atomic emission spectrometer (ICP-AES) evidences the change of Mn concentration in the electrolyte (Supplementary Fig. 11 ; Supplementary Note 1 ). On discharging, the amount of dissolved Mn increases and corresponds to ~ 8.9% of the total manganese at full discharge. The partial dissolution of Mn in electrolyte is a feasible attribution to the noticeable capacity loss on cycling. Fig. 4 XAS characterization of β-MnO 2 electrode. a Mn-K edge XANES curves at selected discharge/charge states, with reference to standard MnO, Mn 2 O 3, and Mn 3 O 4 . b Fitted linear relationship between the photon energy and oxidation state of Mn element. c The EXAFS spectra. d Schematic depiction of the unit cell of β-MnO 2 Full size image Figure 4c shows the EXAFS (extended X-ray absorption fine structure) spectra of β-MnO 2 electrode at selected Zn (de)intercalation stages. The strongest peak located at 1.5 Å is attributed to the closest oxygen (Mn-O) in the MnO 6 octahedra. The peaks at 2.5 and 3.0 Å are assigned to Mn in the edge-sharing (Mn-Mn edge ) and corner-sharing (Mn-Mn corner ) MnO 6 octahedra (Fig. 4d ), respectively [51] , [54] . When the elcctrode was fully discharged, the relative intensity of the Mn-Mn corner peak decreased to a much larger extent than that of Mn-O and Mn-Mn edge signals (Supplementary Fig. 12 ). This result is indicative of the breakage of the corner-shared MnO 6 octahedra. Furthermore, the 3.0 Å peak broadens and slightly shifts to larger distance, which is related to the formation of Mn-O-Zn energy-absorbing path between the layered MnO 6 octohedron slabs and inserted Zn ions. A comparison of the crystallographic structure between β-MnO 2 and Zn-buserite suggests that the co-insertion of Zn 2+ and H 2 O and the dissolution of Mn distort the pyrolusite framework, leaving Mn vacancies in the upper/underlying layers and generating layered Zn-buserite. This tunnel-to-layer phase transition is irreversible, as indicated by the absence of EXAFS spectra recovery on first recharge. Meanwhile, the broadened 3.0 Å peak is not fully recovered after second charging, which can be attritubed to the capacity loss (Fig. 2b ). Notably, XAS analysis of α-MnO 2 and γ-MnO 2 electrodes (Supplementary Fig. 13 ) reveals similar behavior with that of β-MnO 2 , again suggesting common electrode reaction mechanism among different tunneled MnO 2 polymorphs. Electrochemical performance To evaluate the electrochemical performance, coin-type Zn-MnO 2 cell was assembled in ambient air by using β-MnO 2 nanorod cathode, Zn foil anode, filter paper separator, and aqueous Zn(CF 3 SO 3 ) 2 electrolyte. The concentrated 3 M Zn(CF 3 SO 3 ) 2 results in better cyclic stability than diluted electrolyte (e.g., 1 M) (Supplementary Fig. 14 ), which is ascribed to the decrease of water activity and water-induced side reactions [4] , [24] , [55] . As shown in Fig. 1c , the cells based on mild acidic electrolye (3 M ZnSO 4 , pH ~ 3.4; 3 M Zn(CF 3 SO 3 ) 2 , pH ~ 3.6) show much better cycling performance as compared with that employing KOH electolyte. Meanwhile, the cell using Zn(CF 3 SO 3 ) 2 electrolyte delivers much higher initial discharge capacity than that of ZnSO 4 (275 vs. 120 mAh g −1 ) at 0.65 C. However, similar capacity deterioration is observed upon cycling, due to the loss of active mass. To address this issue, we pre-added Mn 2+ salts into the electrolyte to accommodate the dissolution equilibrium of Mn 2+ from MnO 2 electrode. By eliminating the anion effect, we selected Mn(CF 3 SO 3 ) 2 as the electrolyte additive, with concentration from diluted 0.01 M to the saturated 0.1 M. The optimized electrolyte composition was found to be 3 M Zn(CF 3 SO 3 ) 2 + 0.1 M Mn(CF 3 SO 3 ) 2 , which results in the highest Coulombic efficiency and ionic conductivity as well as high capacity of 225 mAh g −1 after 100 cycles (Supplementary Figs. 15 and 16 ). Figure 5a shows the charge/discharge profiles of Zn-MnO 2 cells at different current densities. 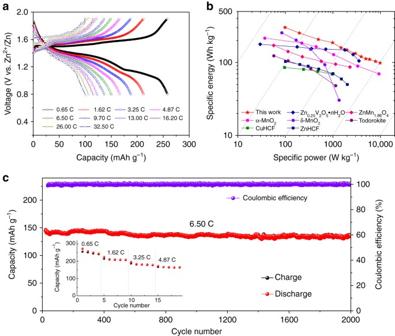Fig. 5 Electrochemical performance of Zn-MnO2cells in 3 M Zn(CF3SO3)2electrolyte with 0.1 M Mn(CF3SO3)2additive.aDischarge/charge profiles at varying C rates.bThe Ragone plots of Zn-MnO2battery and ZIBs with other reported cathode materials. Values are based on the total active mass of both cathode and anode.cLong-cycle performance at rate of 6.5 C.Insetshows the capacity evolution at the initial 19 cycles Discharge capacities of 258, 213, 188, 151, and 115 mAh g −1 were recorded at rates of 0.65, 1.62, 3.25, 6.50, and 16.20 C, respectively. Even at a high rate of 32.50 C, a reversible capacity of 100 mAh g −1 could be obtained. In addition, when the rate shifted back to 0.65 C, the capacity recovered to 246 mAh g −1 , showing a strong tolerance to the rapid Zn 2+ ions insertion/extraction (Supplementary Fig. 17 ). The superior rate performance can be further viewed from the Ragone plots (specific energy vs. specific power) by comparing the Zn-MnO 2 system to reported α-MnO 2 [33] , δ-MnO 2 [56] , Zn 0.25 V 2 O 5 ·nH 2 O [9] , Zn 1.86 Mn 2 O 4 [24] , todorokite [37] , KCuFe(CN) 6 (CuHCF) [21] , and Zn 3 [Fe(CN) 6 ] 2 (ZnHCF) [57] cathodes for aqueous ZIBs (Fig. 5b ). High-specific energy and specific power (254 Wh kg −1 at 197 W kg −1 ; 110 Wh kg −1 at 5910 W kg −1 ) can be simultaneously achieved, which is promising for energy storage applications. The Zn-MnO 2 cell was galvanostatically discharged/charged at 6.50 C (Fig. 5c ) to evaluate the long-term cycling stability. Remarkably, the reversible capacity sustains 135 mAh g −1 with a capacity retention of 94% over 2000 cycles and Coulombic efficiency approaching 100%. Fig. 5 Electrochemical performance of Zn-MnO 2 cells in 3 M Zn(CF 3 SO 3 ) 2 electrolyte with 0.1 M Mn(CF 3 SO 3 ) 2 additive. a Discharge/charge profiles at varying C rates. b The Ragone plots of Zn-MnO 2 battery and ZIBs with other reported cathode materials. Values are based on the total active mass of both cathode and anode. c Long-cycle performance at rate of 6.5 C. Inset shows the capacity evolution at the initial 19 cycles Full size image We also investigated the Zn-MnO 2 cells with 3 M ZnSO 4 + 0.1 M MnSO 4 and 3 M Zn(CF 3 SO 3 ) 2 + 0.1 M MnSO 4 electrolytes, which delivered initial discharge capacity of 110 and 205 mAh g −1 , respectively (Supplementary Fig. 18 ). In SO 4 2− -based electrolyte, an increase of capacity was observed within the first several cycles, which was attributed to the activation process that has been similarly found in reported α-/γ-MnO 2 cathodes [34] , [35] , [36] . Interestingly, the CF 3 SO 3 − -based electrolyte endows much higher initial discharge capacity (275 mAh g −1 at 0.65 C) and results in capacity stabilization after ~ 10 cycles. The different behaviors could be ascribed to the Zn(CF 3 SO 3 ) 2 solution that not only features higher ionic conductivity (Supplementary Fig. 19 ) but also enables faster kinetics and higher stability of Zn plating/stripping as compared with sulfate and alkaline electrolytes (Supplementary Fig. 20 ; Supplementary Note 2 ). Besides, the bulky CF 3 SO 3 − anion (vs. SO 4 2− with double charge) could decrease the number of water molecules surrounding Zn 2+ cations and reduce the solvation effect [24] , thus facilitating Zn 2+ ions transportation and charge transfer. Although the pre-addition of Mn 2+ in electrolyte has been demonstrated to enhance the cyclability of MnO 2 electrode [35] , the underneath mechanism remains unclear. 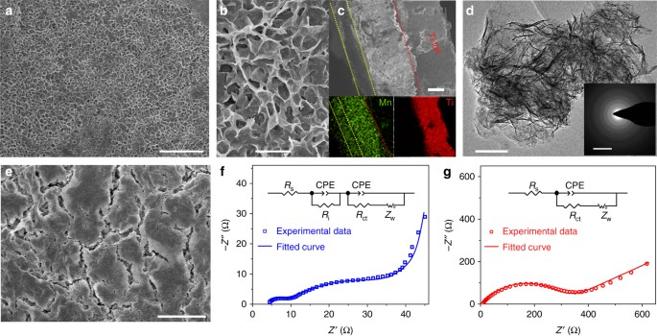Fig. 6 Function of pre-added Mn2+in electrolyte.a,b,c,eSEM,dTEM images, andf,gthree-electrode-cell EIS analysis of re-obtained cathodes after ten cycles in 3 M Zn(CF3SO3)2electrolytea–d,fwith ande,gwithout 0.1 M Mn(CF3SO3)2additive.Insetsofc,dshow elemental mapping and SAED pattern, respectively.Insetsoff,gshow the equivalent circuit to fit the EIS data, whereRs,Ri,Rct, CPE, andZwrepresent series resistance, interface resistance between electrolyte and deposited layer, charge-transfer resistance, constant-phase element, and Warburg diffusion process, respectively.Scale bars, 5 μma,e; 1 μmb; 10 μmc; 100 nmd; and 5 1/nm (insetofd), respectively To further understand the functions of pre-added Mn 2+ , we have carried out a series of analytical studies, including electrochemical measurements, XRD, Raman, XPS, XANES, and SEM/TEM. In acidic electrolyte, manganese oxides (MnO x ) such as MnO 2 or Mn 2 O 3 can be generated from electrolysis of Mn 2+ -containing solution [32] based on the following reactions: 
    MnO_2 + 4H^ +  + 2e^ -  = Mn^2 +  + 2H_2O  
    E^θ = 2.01  V( vs.  Zn^2 + /Zn)
 (1) 
    Mn_2O_3 + 6H^ +  + 2e^ -  = 2Mn^2 +  + 3H_2O  
    E^θ = 2.26  V( vs.  Zn^2 + /Zn)
 (2) According to Nernst equation, the required theoretical potentials to form MnO 2 and Mn 2 O 3 in Mn(CF 3 SO 3 ) 2 (0.1 M, pH 6.0) solution are 1.35 and 1.26 V (vs. Zn 2+ /Zn), respectively; the corresponding values are 1.60 and 1.64 V in 3 M Zn(CF 3 SO 3 ) 2 electrolyte containing 0.1 M Mn 2+ (pH 3.8). This estimation is consistent with the voltammetry results of three-electrode measurements (Supplementary Fig. 21 ; Supplementary Note 3 ), which also reveals that Mn 2+ is not reduced within the investigated potential windows. After charging in 3 M Zn(CF 3 SO 3 ) 2 + 0.1 M Mn(CF 3 SO 3 ) 2 electrolyte, brown deposit layer was observed on the electrode. The layer is composed of manganese oxide with Mn oxidation state between + 3 and + 4, and features nanosheet morphology and poor crystallinity, as analyzed by SEM, XRD, Raman, XPS, and XAENS (Supplementary Fig. 22 ). In post-mortem analysis of Zn-MnO 2 cell using 3 M Zn(CF 3 SO 3 ) 2 + 0.1 M Mn(CF 3 SO 3 ) 2 electrolyte, we also observed an interconnected porous MnO x layer on the cathode surface after charging (Fig. 6a, b ). The cross-sectional SEM image and elemental mapping images (Fig. 6c ) evidence the presence of a uniform layer with thickness around 10 μm. TEM imaging and selected area electron diffraction (SAED) analysis reveal porous nanosheet microstructure and amorphous character of the deposited layer (Fig. 6d ), which would facilitate mass diffusion. In contrast, the integrity of β-MnO 2 electrode was seriously destroyed with the formation of cracks in 3 M Zn(CF 3 SO 3 ) 2 electrolyte without Mn(CF 3 SO 3 ) 2 additive (Fig. 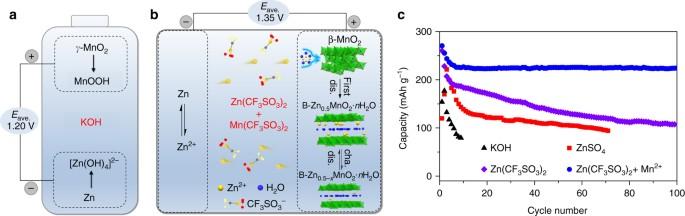6e ). The electrode pulverization would break the electronic conducting network and increase electrode polarization, further aggravating the capacity decay. Electrochemical impedance spectroscopy (EIS) was performed in a three-electrode cell, using the dismantled cathode after ten cycles as the working electrode, platinum plate as the counter electrode, and saturated calomel electrode (SCE) as the reference electrode. The cycled electrode in Mn 2+ -added electrolyte displays two depressed semicircles in high frequency area and one line in low frequency region (Fig. 6f ). Fig. 1 Zn-MnO2battery chemistry. Schematic illustration ofathe primary alkaline Zn-MnO2battery using KOH electrolyte andbthe rechargeable Zn-MnO2cell using CF3SO3−-based electrolyte.cComparison of the cycling performance of Zn-MnO2cells with electrolytes of 45wt.% KOH (at 0.32 C), 3 M ZnSO4, 3 M Zn(CF3SO3)2, and 3 M Zn(CF3SO3)2with 0.1 M Mn(CF3SO3)2additive at 0.65 C.nC equals the rate to charge/discharge the thereotical capacity (308 mAh g−1) of MnO2in 1/nhours Fitting the EIS data (Supplementary Table 1 ) gives a series resistance ( R s , 4.5 Ω), an interface resistance ( R i , 6.0 Ω) between electrolyte and deposited layer, a charge-transfer resistance ( R ct , 25 Ω) and a Warburg diffusion impedance ( Z w , 124.7 Ω). In comparison, the cell without electrolyte additive shows higher R s (8.0 Ω), R ct (350 Ω), and Z w (1200 Ω), in the absence of the apparent interface component (Fig. 6g ). Fig. 6 Function of pre-added Mn 2+ in electrolyte. a , b , c , e SEM, d TEM images, and f , g three-electrode-cell EIS analysis of re-obtained cathodes after ten cycles in 3 M Zn(CF 3 SO 3 ) 2 electrolyte a – d , f with and e , g without 0.1 M Mn(CF 3 SO 3 ) 2 additive. Insets of c , d show elemental mapping and SAED pattern, respectively. Insets of f , g show the equivalent circuit to fit the EIS data, where R s , R i , R ct , CPE, and Z w represent series resistance, interface resistance between electrolyte and deposited layer, charge-transfer resistance, constant-phase element, and Warburg diffusion process, respectively. Scale bars , 5 μm a , e ; 1 μm b ; 10 μm c ; 100 nm d ; and 5 1/nm ( inset of d ), respectively Full size image Based on the above results, we propose three merits of the Mn 2+ electrolyte additive for the Zn-MnO 2 battery: (1) accommodating and compensating Mn 2+ dissolution from the electrode, (2) improving initial Coulombic efficiency and ionic conductivity of the electrolyte and (3) generating a uniform porous nanostructured MnO x film on the cathode surface, which helps to maintain the electrode integrity and favor charge transfer. Note that the generated MnO x layer itself contributes to nearly 2.4% of the capacity delivered by the active material (Supplementary Fig. 23 ). The Zn(CF 3 SO 3 ) 2 + Mn(CF 3 SO 3 ) 2 electrolyte is also applicable to improve the cycling stability of nanostructured α-MnO 2 and γ-MnO 2 cathodes (Supplementary Fig. 24a, b ). Furthermore, commercial β-MnO 2 powders with irregular shape and micrometer particle size (Supplementary Fig. 3 ) also exhibit considerable capacity (132 mAh g −1 at 0.65 C) and cyclability (200 cycles) in this electrolyte (Supplementary Fig. 24c, d ). The Zn anode was also investigated to understand the high-performing Zn-MnO 2 cell chemistry (Supplementary Figs. 25 – 28 ). Post-mortem analysis of cycled Zn in three-electrode cell with 3 M Zn(CF 3 SO 3 ) 2 + 0.1 M Mn(CF 3 SO 3 ) 2 electrolyte reveals a dense and dendrite-free surface morphology after 280 h of repeated Zn plating/stripping (Supplementary Fig. 25 ). In a Zn-MnO 2 full cell, neither dendritic morphology nor formation of byproducts such as ZnO or Zn(OH) 2 was evidenced after rate test (Supplementary Fig. 26 ), favoring the cyclic stability of Zn-MnO 2 batteries. In contrast, in 3 M ZnSO 4 + 0.1 M MnSO 4 electrolyte, Zn plate with lots of cracks formed on the zinc surface, while ZnO nanorods were observed in KOH electrolyte, which would deter the cyclability of Zn (Supplementary Figs. 25 and 27 ). Furthermore, the EDS analysis indicates that there is no detectable Mn in Zn anode (Supplementary Fig. 28 ). The exceptional performance of Zn-MnO 2 coin-type batteries has motivated us to further assess soft-packed full cells, which were facilely assembled in ambient air negating complicated procedures or extra protection ( Supplementary Methods ). 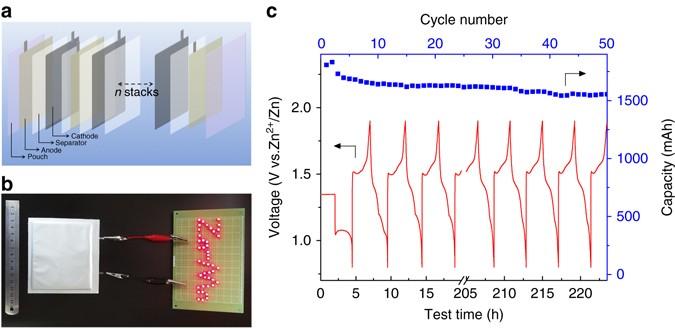Fig. 7 Electrochemical performance of pouch-type Zn-MnO2battery.aSchematic illustration of the cell configuration with anode—separator—cathode stacks.bA digital photo of the soft-package battery powering a series of LED lights.cCycling performance in the voltage range of 0.8–1.9 V at constant current of 0.72 A Figure 7a schematically shows the battery configuration consisting of six anode—separator—cathode stacks. A typical assembled pouch-type cell lightens a “Zn-Mn”—shape indicator containing 44 LEDs (Fig. 7b ). A stable discharge capacity of 1550 mAh can be obtained after 50 repeated cycles with an average potential of 1.35 V (Fig. 7c ). The full cell delivers an energy density of 158.5 Wh kg −1 based on the total weight of the active materials (including both cathode and anode). This value far exceeds that of other aqueous Li-ion batteries (50–90 Wh kg −1 ) [3] , [4] , [58] and aqueous Na-ion batteries (~ 33 Wh kg −1 ) [8] , [16] , [59] . Remarkably, a total energy density of 75.2 Wh kg −1 is obtained according to the mass of whole battery mass, much higher than that of commercial Pb-acid (~ 30 Wh kg −1 ) and Ni-Cd technologies (~ 50 Wh kg −1 ) [26] . We note that the higher price of anhydrous Zn(CF 3 SO 3 ) 2 salt relative to ZnSO 4 and KOH would inevitably increase the practical cost of this aqueous Zn-MnO 2 battery system, even though Zn(CF 3 SO 3 ) 2 merely serves as charge carrier and is not consumed during battery operation. Fortunately, considering the abundant, cheap precursors (i.e., triflic acid and ZnCO 3 ) [60] and the direct usage of hydrate-form salt in aqueous solution, the cost of Zn(CF 3 SO 3 ) 2 electrolyte could be expected to drop with the development of synthetic technique and market demand. Fig. 7 Electrochemical performance of pouch-type Zn-MnO 2 battery. a Schematic illustration of the cell configuration with anode—separator—cathode stacks. b A digital photo of the soft-package battery powering a series of LED lights. c Cycling performance in the voltage range of 0.8–1.9 V at constant current of 0.72 A Full size image In conclusion, we demonstrate a high-performing rechargeable Zn-MnO 2 battery system based on zinc anode, β-MnO 2 cathode, and mild acidic aqueous electrolyte. We elucidate the Zn-insertion mechanism and structural evolution of MnO 2 cathode by combining electrochemical investigations, XRD, TEM, ICP, and XANES/EXAFS analysis. A phase transition from tunneled to layered structure (Zn-buserite) occurs during the first discharge of MnO 2 , followed by reversible Zn 2+ (de)intercalation in the H 2 O-containing Zn-buserite framework. Unlike previous reports, this electrode mechanism is common in polymorphs of α-MnO 2 , γ-MnO 2 , and β-MnO 2 . The phase tranformation, Mn dissolution and electode pulverization incur capacity fade of MnO 2 . By formulating an aqueous 3 M Zn(CF 3 SO 3 ) 2 + 0.1 M Mn(CF 3 SO 3 ) 2 electrolyte, the Mn 2+ dissolution can be effectively accommodated and the electrode integrity can be maintained because of the in-situ generated amorphous MnO x layer. As a result, Zn-MnO 2 cell exhibits high capacity (225 mAh g −1 at 0.65 C), high rate capability (100 mAh g −1 at 32.50 C) and long-term cycling stability (94% capacity retention after 2000 cycles at 6.50 C). Furthermore, the assembled soft-packed Zn-MnO 2 battery can deliver a high reversible capacity of 1550 mAh with a total energy density of 75.2 Wh kg −1 , among the highest value achieved in aqueous battery technologies. The present Zn-MnO 2 system holds great promise for potential applications in large-scale energy storage, in view of the remarkable electrochemical performance and other advantages such as low materials cost, easy manufacturing, high safety, and environmental friendliness. Synthesis β-MnO 2 nanorods were synthesized by a hydrothermal method. In a typical synthesis, 30 ml KMnO 4 (0.1 M) and 30 ml MnSO 4 ·H 2 O (0.6 M) were mixed under continuous stirring for 30 min at room temperature. The mixture was loaded into a 100 ml Teflon-lined autoclave and maintained at 140 °C for 12 h. The obtained product was centrifuged, washed thoroughly using water and absolute ethyl alcohol, and dried at 80 °C for 10 h. Bulk β-MnO 2 powders was purchased from Alfa Aesar . α-MnO 2 and γ-MnO 2 nanorods were synthesized via hydrothermal technique following previously reported procedures [61] . Characterization Powder XRD patterns were collected on a Rigaku X-ray diffractometer (MiniFlex600) with Cu Kα radiation. SEM images were obtained on Field-emission JEOL JSM-7500F microscope. TEM and HRTEM images were taken on Philips Tecnai G2 F20. ABF-STEM was performed on Titan Cubed Themis G2 300 (FEI) at an acceleration voltage of 200 kV. The XAS data were collected on BL14W1 beamline of Shanghai Synchrotron Radiation Facility and analyzed with software of Ifeffit Athena [62] . ICP-AES measurements were conducted on a PerkinElmer Optima 8300. XPS was tested on a Perkin Elmer PHI 1600 ESCA system. Raman spectra were obtained on confocal Thermo-Fisher Scientific DXR microscope using 532 nm excitation. TGA was measured by a Netzsch STA 449 F3 Jupiter analyzer. Electrochemical test Electrochemical performance was tested using CR2032 coin-type cells. The working electrode was fabricated by blending MnO 2 powder, Super P carbon and polyvinylidene fluoride in a weight ratio of 8:1:1 using N -methyl-2-pyrrolidone as solvent. The obtained slurry was pasted onto a Ti foil and vacuum-dried at 100 °C for 12 h. The loading mass of active material was ~ 2 mg cm −2 . Filter paper and zinc foil were employed as the separator and anode, respectively. A 3 M Zn(CF 3 SO 3 ) 2 with/without 0.1 M Mn(CF 3 SO 3 ) 2 aqueous solution was used as the electrolyte. The assembled cells were galvanostatically cycled between 0.8 and 1.9 V using the LAND-CT2001A battery-testing instrument. Calculation of specific capacities was based on the mass of initial MnO 2 . CVs were measured on a Parstat 263 A electrochemical workstation (AMETEK). EIS was performed on a Parstat 2273 electrochemical workstation (AMETEK). The AC perturbation signal was ± 10 mV and the frequency ranged from 100 kHz to 100 mHz. The electrochemical behaviors of Mn 2+ additive in electrolyte were characterized using three-electrode cells (Ti foil as working electrode, platinum plate or Zn foil as counter electrode, and SCE as reference electrode). Data availability The authors declare that all the relevant data are available within the paper and its Supplementary Information file or from the corresponding author upon reasonable request.